Phosphorescent dye-based supramolecules for high-efficiency organic light-emitting diodes Organic light-emitting diodes (OLEDs) are among the most promising organic semiconductor devices. The recently reported external quantum efficiencies (EQEs) of 29–30% for green and blue phosphorescent OLEDs are considered to be near the limit for isotropically oriented iridium complexes. The preferred orientation of transition dipole moments has not been thoroughly considered for phosphorescent OLEDs because of the lack of an apparent driving force for a molecular arrangement in all but a few cases, even though horizontally oriented transition dipoles can result in efficiencies of over 30%. Here we use quantum chemical calculations to show that the preferred orientation of the transition dipole moments of heteroleptic iridium complexes (HICs) in OLEDs originates from the preferred direction of the HIC triplet transition dipole moments and the strong supramolecular arrangement within the co-host environment. We also demonstrate an unprecedentedly high EQE of 35.6% when using HICs with phosphorescent transition dipole moments oriented in the horizontal direction. The efficiency of light emission from organic light-emitting diodes (OLEDs) is one of their most important characteristics, along with emission colour and lifetime, because it is directly related to power consumption and device longevity. External quantum efficiencies (EQEs) of 30% have been reported recently [1] , [2] , [3] , [4] , [5] , [6] ; this is considered to be the light-outcoupling efficiency limit of phosphorescent OLEDs under isotropically oriented transition dipole moments [4] . It has long been recognized that orienting the transition dipole moment of an emitter along the horizontal direction (parallel to the substrate) can enhance the outcoupling efficiency beyond that achieved under isotropic orientation, as demonstrated in polymer-based and vacuum-evaporated fluorescent molecule-based OLEDs [7] , [8] , [9] , [10] , [11] , [12] , [13] . Nonetheless, the orientation of the transition dipole moments of iridium complexes used as phosphorescent emitters in efficient OLEDs is typically considered to be isotropic because they are near-globular and small enough to have configurational diversity in their orientational states. Therefore, it is believed that the theoretical EQE limit of phosphorescent OLEDs is 30%. Recently, however, some heteroleptic iridium complexes (HICs) have been reported to have transition dipole moments oriented preferentially along the horizontal direction [5] , [14] , [15] , [16] , [17] , [18] . This implies that it may be possible to exceed the efficiency limit of 30% under isotropic orientations of the emitting dipoles. Unfortunately, the origin of the preferred orientation of some phosphorescent dyes is not fully understood, and OLEDs with an EQE over 30% have not yet been demonstrated using oriented phosphorescent dyes. In this article, we use quantum chemical calculations to show that the heteroleptic structure and the strong intermolecular interactions between HICs and their host molecules lead to preferred dipole orientations in the HICs. We demonstrate an unprecedentedly high EQE of 35.6% for red-emitting HICs with triplet transition dipole moments oriented along the horizontal direction. Materials for OLEDs The red-emitting HICs Ir(mphq) 2 acac [(bis(2-(3,5-dimethylphenyl)quinoline)Ir(III)(acetylacetonate)] [19] , Ir(MDQ) 2 acac [bis(2-methyldibenzo-[ f , h ]-quinoxaline)Ir(III)(acetylacetonate)] [20] and Ir(mphmq) 2 tmd [(bis(4-methyl-2-(3,5-dimethylphenyl)quinoline))Ir(III)(tetramethylheptadionate)] [19] were used as phosphorescent emitters, and N , N ′-di(naphthalen-1-yl)- N , N ′-diphenylbenzidine (NPB) and bis(4,6-(3,5-di-(3-pyridyl)phenyl))-2-methylpyrimidine (B3PYMPM) were used as co-hosts for the fabrication of the OLEDs. A reference complex ( fac -Ir(phq) 3 ) [21] with a homoleptic disposition of the ligands identical to those of Ir(mphq) 2 acac was also prepared. The chemical structures of the red-emitting dyes and the host materials are presented in Fig. 1a . The photoluminescence (PL) quantum yields ( q PL ’s) of the emitting layers (EMLs) were directly measured using 50-nm-thick films on quartz substrates in an integration sphere. The measured q PL ’s of the dyes were 0.71 for fac -Ir(phq) 3 , 0.83 for Ir(mphq) 2 acac, 0.82 for Ir(MDQ) 2 acac and 0.96 for Ir(mphmq) 2 tmd. The co-host system was selected to take advantage of its exciplex-forming characteristics because OLEDs containing an exciplex-forming co-host have an almost perfect electron-hole balance, low driving voltage and low efficiency roll-off [1] , [5] , [22] , [23] . 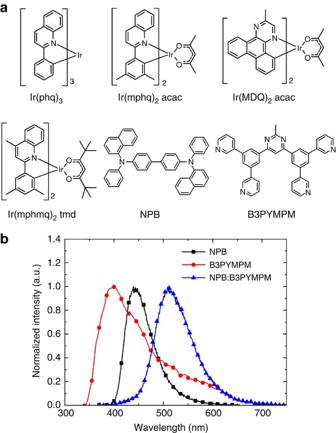Figure 1: Material characteristics. (a) Molecular structures of the red phosphorescent dyes and the host molecules. (b) Normalized PL spectra of the NPB, B3PYMPM and mixed NPB:B3PYMPM films. Figure 1b shows the PL spectra of vacuum-evaporated films of NPB and B3PYMPM and a co-evaporated film of NPB and B3PYMPM with a molar ratio of 1:1. The co-evaporated film exhibits featureless emission at 510 nm that is red-shifted compared with those of its constituent materials. The peak wavelength is close to the energy difference between the energy levels of the lowest unoccupied molecular orbital (LUMO) of B3PYMPM and the highest occupied molecular orbital (HOMO) of NPB, indicating that the co-host system efficiently forms exciplexes upon photoexcitation. Figure 1: Material characteristics. ( a ) Molecular structures of the red phosphorescent dyes and the host molecules. ( b ) Normalized PL spectra of the NPB, B3PYMPM and mixed NPB:B3PYMPM films. Full size image Orientations of transition dipole moments of the phosphorescent dyes The orientations of the transition dipole moments of the red dyes in the mixed co-host films were determined by analysing the angle-dependent PL spectra of the films [5] , [12] , [13] , [15] . The birefringence of the EML was considered in the theoretical fittings. 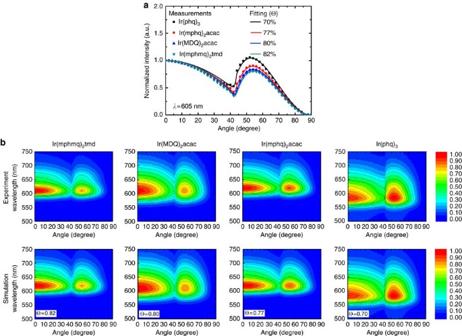Figure 2: Analysis of the orientations of the transition dipole moments. (a) Angle-dependent PL intensities at 605 nm and (b) angle-dependent PL spectra ofp-polarized light from the 30-nm-thick NPB:B3PYMPM:red dye (0.5:0.5:0.035 molar ratio) film. The theoretical calculations fit the experimental data well. Figure 2a shows the measured angle-dependent PL intensities of the p -polarized light emitted from the 30-nm-thick NPB:B3PYMPM:red dye (0.48:0.48:0.035 molar ratio) films at 605 nm, which are close to the PL maxima of the red emitters. The experimental data fit the horizontal transition dipole ratios (Θ’s) of 0.70 for fac -Ir(phq) 3 , 0.77 for Ir(mphq) 2 acac, 0.80 for Ir(MDQ) 2 acac and 0.82 for Ir(mphmq) 2 tmd with an uncertainty of ±2%, where Θ is defined as the ratio of the horizontal component of the transition dipole moments to the total transition dipole moments. Moreover, the angle-dependent PL spectra were well matched, with theoretical fittings at all wavelengths ( Fig. 2b ). Fac -Ir(phq) 3 , a homoleptic iridium complex, exhibited nearly isotropically oriented transition dipole moments, whereas the transition dipoles of the HICs were preferentially oriented along the horizontal direction, as manifested by the Θ values of over 0.75. Figure 2: Analysis of the orientations of the transition dipole moments. ( a ) Angle-dependent PL intensities at 605 nm and ( b ) angle-dependent PL spectra of p -polarized light from the 30-nm-thick NPB:B3PYMPM:red dye (0.5:0.5:0.035 molar ratio) film. The theoretical calculations fit the experimental data well. Full size image Two conditions should be satisfied to obtain transition dipole moments preferentially oriented in the horizontal direction in the red HIC-doped co-host films: (1) the HIC should have triplet transition dipole moments preferentially oriented along a specific direction and not have a combination of transition dipole moments with various orientations, and (2) the HIC molecule itself should have a preferred orientation with respect to the substrate, in such a way that the combination of both conditions leads to transition dipole moments that are parallel to the horizontal direction. To determine the detailed mechanism for (1) and (2), molecular simulations were performed. The triplet-state geometries of the red dyes were calculated using an unrestricted B3LYP level of theory without symmetry constraints. The triplet-state geometries of the HICs were found to possess a molecular C 2 axis that intersected the iridium core and the central carbon atom of the β-diketonate ancillary ligand. The pseudo octahedral geometry was completed by the remaining phenylato parts of the main ligands, which were located along the diagonal lines that cross the oxygen atom and the iridium core. In the case of fac -Ir(phq) 3 , the triplet-state geometry adopted C 3 symmetry. Inspection of the Kohn–Sham orbitals revealed that the HOMO was distributed over the d( t 2g )-orbital of Ir(III) and the π-orbital of the phenylato moiety, whereas the LUMO was mainly localized in the π*-orbital of the N -heterocycles ( Fig. 3a ). Time-dependent density functional theory (TD−DFT) calculations were subsequently carried out for the optimized geometries to determine their adiabatic triplet transition energies, and these were found to be 1.81 eV for fac -Ir(phq) 3 , 1.79 eV for Ir(mphq) 2 acac, 1.86 eV for Ir(MDQ) 2 acac and 1.83 eV for Ir(mphmq) 2 tmd. In each case, the triplet transition mainly comprised an electronic transition from the HOMO to the LUMO with a configuration interaction coefficient larger than 0.62. The triplet transition dipole moment was calculated using the quadratic response function [24] , [25] . 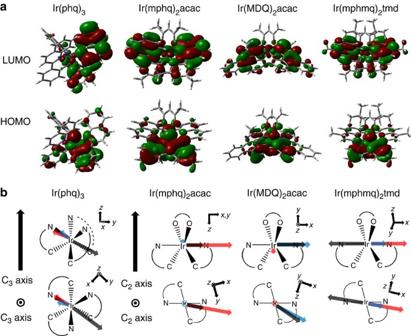Figure 3: Quantum chemical calculations of the red dyes based on DFT. (a) Frontier molecular orbitals contributing to the lowest triplet transitions of Ir(phq)3, Ir(mphq)2acac, Ir(MDQ)2acac and Ir(mphmq)2tmd. (b) The triplet transition dipole moments of Ir(phq)3, Ir(mphq)2acac, Ir(MDQ)2acac and Ir(mphmq)2tmd from three spin sublevels are shown as arrows. The transition dipole moments of theTx,TyandTzsublevels correspond to the black, red and blue arrows respectively. Figure 3b shows the x , y , z directions of the dipole moment for the transition from three sublevels of the triplet state. The angles between the C 2 axis and the direction of the total triplet transition dipole moments of the HICs were found to be nearly right angles, with values of 89.02° for Ir(mphq) 2 acac, 85.19° for Ir(MDQ) 2 acac and 90.45° for Ir(mphmq) 2 tmd. In sharp contrast, the directions of the triplet transition dipole moments of fac -Ir(phq) 3 adopted a slant angle of 67.6° with respect to the C 3 axis. Therefore, the axial components ( ⊥ ) of the transition dipole moments along the C 3 axis were approximately half of the equatorial components ( ‖ ) in the molecule ( ‖ : ⊥ =2.4:1). The full calculation results, including the individual values of the transition dipole moments, are summarized in Supplementary Table 1 . Figure 3: Quantum chemical calculations of the red dyes based on DFT. ( a ) Frontier molecular orbitals contributing to the lowest triplet transitions of Ir(phq) 3 , Ir(mphq) 2 acac, Ir(MDQ) 2 acac and Ir(mphmq) 2 tmd. ( b ) The triplet transition dipole moments of Ir(phq) 3 , Ir(mphq) 2 acac, Ir(MDQ) 2 acac and Ir(mphmq) 2 tmd from three spin sublevels are shown as arrows. The transition dipole moments of the T x , T y and T z sublevels correspond to the black, red and blue arrows respectively. Full size image The molecular arrangements and orientations of the red emitters with respect to the underlying substrate in the EML also influenced the orientation of the transition dipole moments. The optical anisotropy with different ordinary and extraordinary refractive indices was measured by variable angle spectroscopic ellipsometry (VASE), and the data indicated that the molecular long axes of the host molecules were parallel to the substrate ( Supplementary Fig. 1 ) [26] . Because the EML contains a small amount of red dyes (~0.035 mol fraction), the molecular orientations of the red dyes and their resultant electro-optic performance rely on the binding geometries of the red dyes with the host molecules. To computationally investigate the intermolecular interactions between the constituent molecules in the EML, geometry optimizations were performed on the NPB/B3PYMPM/red dye ternary systems using DFT with the Perdew–Burke–Ernzerhof functional [27] with a double numerical basis set and the polarization basis set under an effective core potential. 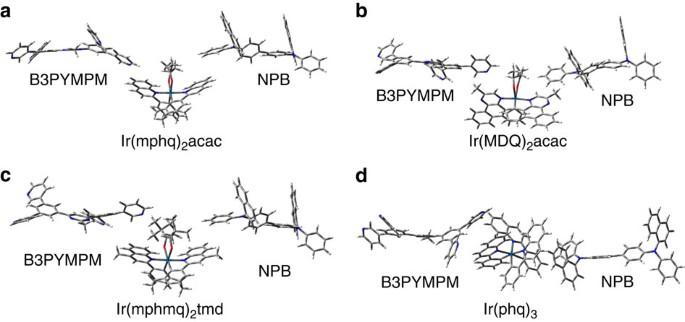Figure 4: Optimized binding geometries of the red dye co-host supramolecules. (a) B3PYMPM-Ir(mphq)2acac-NPB, (b) B3PYMPM-Ir(MDQ)2acac-NPB, (c) B3PYMPM-Ir(mphmq)2tmd-NPB and (d) B3PYMPM-Ir(phq)3-NPB. Figure 4a–d shows the optimized geometries of the red dye/co-host molecular clusters (or supramolecules), revealing that the C 2 axis of the HICs (Ir(mphq) 2 acac, Ir(MDQ) 2 acac and Ir(mphmq) 2 tmd), as well as the C 3 axis of fac -Ir(phq) 3 were almost perpendicular to the molecular long axes of the NPB and B3PYMPM molecules. The binding energies of the four red dye/co-host systems (that is, NPB−dye−B3PYMPM) were almost identical at ~70 kcal mol −1 . The pairwise binding energies of the NPB/B3PYMPM/dye systems are given in Table 1 . Notably, the binding energies between the HICs and the host molecules (NPB or B3PYMPM) were ~10−20 times stronger than the binding energies between the other binding pairs (2−3 kcal mol −1 ). The strong binding energies of the HICs with the host molecules can be attributed mainly to the electron-deficient nature of the N -heterocycles that interact strongly with the electron-rich region of the aromatic rings in the tail of the host molecules. Isosurfaces of the molecular electrostatic potential (ESP) for the HICs and the host molecules are shown in Fig. 5a–f . The isosurfaces suggest that the highly electropositive spots (+0.1 J C −1 ) at the methyl groups (Ir(mphmq) 2 tmd and Ir(MDQ) 2 acac) or hydrogens (Ir(mphq) 2 acac) belonging to the N -heterocycles of the HICs are responsible for the strong Coulomb interactions with the electronegative aromatic planes of the host molecules. From the optimized binding geometries in Fig. 4a–c , the host molecules are docked in the space between these two spots ( N -heterocycles and β-diketonate ancillary ligands), and these are almost perpendicular to the C 2 axes of the HICs. The spaces between the highly electropositive spots can thus be regarded as binding sites for the HIC molecules that lead to supramolecular assembly between the HICs and the host molecules. Because the NPB and B3PYMPM molecules are horizontally oriented in the co-host films, the C 2 axes of the HIC molecules tend to be more or less perpendicular to the film surface. Therefore, it is inferred from these calculations that the preferred orientation of the transition dipole moments of the HICs in the EMLs is along the horizontal direction because of the almost perpendicular direction of the transition dipole moments to the C 2 axis in the HICs. However, a smaller horizontal transition dipole moment is predicted for fac -Ir(phq) 3 because the molecule has a horizontal-to-vertical transition dipole moment ratio of ~0.705:0.295 from the ‖ : ⊥ =2.4:1 because the C 3 axis is perpendicular to the substrate. The ratio is very close to the experimentally obtained Θ=0.70. Notably, the rotation of the homoleptic molecule does not significantly change the orientational factor Θ because of the molecular symmetry. Figure 4: Optimized binding geometries of the red dye co-host supramolecules. ( a ) B3PYMPM-Ir(mphq) 2 acac-NPB, ( b ) B3PYMPM-Ir(MDQ) 2 acac-NPB, ( c ) B3PYMPM-Ir(mphmq) 2 tmd-NPB and ( d ) B3PYMPM-Ir(phq) 3 -NPB. Full size image Table 1 Pairwise binding energies of the hosts (NPB and B3PYMPM) and the red dyes (Ir(phq) 3 , Ir(mphq) 2 acac, Ir(MDQ) 2 acac and Ir(mphmq) 2 tmd). 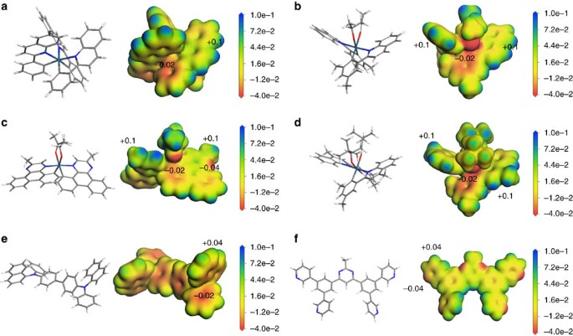Figure 5: Isosurfaces of the molecular ESP. (a) Ir(phq)3, (b) Ir(mphq)2acac, (c) Ir(MDQ)2acac, (d) Ir(mphmq)2tmd, (e) NPB and (f) B3PYMPM. The numerals on the isosurfaces are in J C−1. The electron-deficient nature of theN-heterocycles and the β-diketonate ancillary ligand interact strongly with the electron-rich region of the aromatic rings in the tail of the host molecules. Full size table Figure 5: Isosurfaces of the molecular ESP. ( a ) Ir(phq) 3 , ( b ) Ir(mphq) 2 acac, ( c ) Ir(MDQ) 2 acac, ( d ) Ir(mphmq) 2 tmd, ( e ) NPB and ( f ) B3PYMPM. The numerals on the isosurfaces are in J C −1 . The electron-deficient nature of the N -heterocycles and the β-diketonate ancillary ligand interact strongly with the electron-rich region of the aromatic rings in the tail of the host molecules. Full size image It is worth commenting that our simulations of the binding geometries were based only on the optimization of three molecules, consisting of one emitter molecule and two host molecules. Nonetheless, because the content of emitters in this amorphous mixture is quite small, and because the emitters investigated in this study have only two binding sites with extremely high binding energies to the host molecules (10–20 times those of the emitter–emitter and host–host interactions), we presume that the host–emitter–host supramolecule is a unit pseudo-molecule comprising the emission layer with excessive host molecules and that its internal geometry is little affected by neighbouring pseudo-molecular units or host molecules. Fabrication and performance of the OLEDs Having verified the preferred horizontal orientation of the HIC transition dipoles, we fabricated OLEDs to examine the influence of the anisotropic dipole alignment. 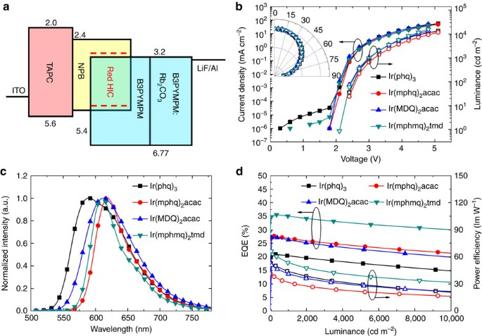Figure 6: Device structure and OLED performance for red dyes. (a) Schematic diagram of the device structure and the energy levels of the device. (b)J–V–Lcurves. Inset: the angular distribution of the EL intensity of the OLEDs. The dashed line in the inset shows the Lambertian distribution. (c) EL spectrum of the OLEDs. (d) EQEs and power efficiency as a function of the luminance. Figure 6a schematically shows the configuration of the device and the energy levels of the layers that were incorporated into the devices. The multilayer OLEDs were prepared with the following layers: indium tin oxide (ITO; 100 nm)/1,1-bis[4-di(p-toluyl)aminophenyl]cyclohexane (TAPC; 75 nm)/NPB (10 nm)/NPB:B3PYMPM: 3.5 mol% red dyes (30 nm)/B3PYMPM (10 nm)/B3PYMPM: 2 wt% Rb 2 CO 3 (45 nm)/Al (100 nm). The NPB and B3PYMPM were used as the hole transport material and the electron transport material, respectively. The hole transport material and electron transport material were also used as co-hosts of the EML at a molar ratio of 1:1. This co-host system facilitates efficient charge injection from the electrodes to the EML because it removes the injection barrier for electrons (or holes) from the electron transport layer (ETL or hole transport layer) to the EML. Figure 6: Device structure and OLED performance for red dyes. ( a ) Schematic diagram of the device structure and the energy levels of the device. ( b ) J – V – L curves. Inset: the angular distribution of the EL intensity of the OLEDs. The dashed line in the inset shows the Lambertian distribution. ( c ) EL spectrum of the OLEDs. ( d ) EQEs and power efficiency as a function of the luminance. Full size image The current density–voltage–luminance ( J – V – L ) characteristics of the OLEDs containing fac -Ir(phq) 3 , Ir(mphq) 2 acac, Ir(MDQ) 2 acac or Ir(mphmq) 2 tmd are shown in Fig. 6b . The devices showed identical J – V characteristics but different L – V characteristics because of the differences in their emission spectra and EQEs. The electroluminescent (EL) spectra ( Fig. 6c ) of the OLEDs matched the PL spectra of the dyes doped in the co-host film well. The EQEs and power efficiencies of the devices calibrated using the profiles of the angle-dependent number of emitted photons (inset of Fig. 6b ) are shown in Fig. 6d . The EQE of the Ir(mphmq) 2 tmd device was higher than that of the devices containing Ir(MDQ) 2 acac, Ir(mphq) 2 acac or fac -Ir(phq) 3 . Specifically, the Ir(mphmq) 2 tmd device showed a very high EQE of 35.6% at a luminance of 350 cd m −2 , which is 1.5 times higher than the highest efficiency reported to date for red OLEDs and even higher than that of green OLEDs [1] , [2] , [3] , [19] , [28] , [29] . The efficiency roll-off was also very small, as the EQE was 35.1% at 1,000 cd m −2 and 30.0% at 10,000 cd m −2 . If one considers the sensitivity of human eyes, red emission with a luminance of 10,000 cd m −2 corresponds to a radiative intensity 2−3 times higher than that of green emission at the same luminance. The high EQE combined with a low turn-on voltage (2.1 V) and a low driving voltage resulted in a high power efficiency with a maximum value of 66.2 lm W −1 (53.6 lm W −1 at 1,000 cd m −2 ) in the optimized device. Optical simulation of the EQE of devices To explain the high EQE, the maximum EQE for the Ir(mphmq) 2 tmd device was simulated as a function of the total thickness of the ETL ( t ETL ) using q PL =0.96 and Θ=0.82 (ref. 30 ). As shown in Fig. 7a , the calculated profiles exhibit a sinusoidal variation in the EQE with increasing t ETL and match the experimental data very well over a wide t ETL range. The J–V–L data, angle-dependent emission patterns, emission spectrum, quantum efficiency and power efficiency data for the devices in Fig. 7a are shown in Supplementary Figs 2–5 . We repeated the calculation of the maximum EQEs of the optimized devices with red dyes using ( q PL , Θ) values of (0.71, 0.70) for fac -Ir(phq) 3 , (0.83, 0.77) for Ir(mphq) 2 acac, (0.82, 0.80) for Ir(MDQ) 2 acac and (0.96, 0.82) for Ir(mphmq) 2 tmd. We assumed a perfect electron-hole balance in these devices. The predicted maximum EQE values for the devices based on fac -Ir(phq) 3 , Ir(mphq) 2 acac, Ir(MDQ) 2 acac and Ir(mphmq) 2 tmd were 22.2%, 29.1%, 29.6% and 34.9%, respectively. These values are in excellent agreement with the measured maximum EQEs of the fac -Ir(phq) 3 (20.9%), Ir(mphq) 2 acac (27.6%), Ir(MDQ) 2 acac (27.1%) and Ir(mphmq) 2 tmd (35.6%) containing devices. The unprecedented value of EQE 35.6% is originated from high Θ combined with high q PL of Ir(mphmq) 2 tmd. 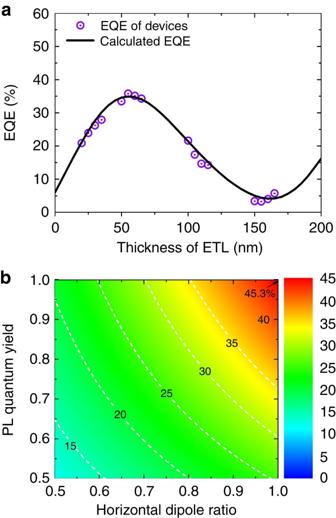Figure 7: Optical simulation of the EQE of devices. (a) EQEs of the Ir(mphmq)2tmd-based OLEDs with varying ETL thickness (circles with dots). TheJ–V–L, angle-dependent emission patterns, emission spectra, quantum efficiencies and power efficiency data for these devices are shown inSupplementary Figs 2–5. (b) Contour plot of the maximum EQEs achievable with Ir(mphmq)2tmd possessing a certain PL quantum yield (qPL) and ratio of the horizontal dipole (Θ). Figure 7: Optical simulation of the EQE of devices. ( a ) EQEs of the Ir(mphmq) 2 tmd-based OLEDs with varying ETL thickness (circles with dots). The J–V–L , angle-dependent emission patterns, emission spectra, quantum efficiencies and power efficiency data for these devices are shown in Supplementary Figs 2–5 . ( b ) Contour plot of the maximum EQEs achievable with Ir(mphmq) 2 tmd possessing a certain PL quantum yield ( q PL ) and ratio of the horizontal dipole (Θ). Full size image Using quantum chemical calculations, we demonstrated that the preferred orientation of HICs in OLEDs originates from the preferred direction of the HIC triplet transition dipole moments and the strong supramolecular arrangement within the co-host environment. The elongated supramolecules themselves or the preferred horizontal orientation of the host molecules resulted in the preferred horizontal triplet transition dipole moments of the HICs in the EML. Understanding the origin of the preferred orientation of HICs will enable us to design dyes with highly oriented transition dipole moments. As a result, it will be possible to achieve EQEs much higher than the conventional limit of 30%. To verify the effect of the orientation of the transition dipole moments on EQE, the simulation was extended to calculate the maximum achievable EQEs for red OLEDs using the emission spectrum of Ir(mphmq) 2 tmd with arbitrary values of q PL and Θ. Figure 7b shows a contour plot of the maximum EQEs for the red OLEDs as a function of q PL and Θ assuming a perfect electron-hole balance without any electrical loss. The figure clearly shows that an EQE of over 45% is achievable if the emitter has a q PL of 1 and horizontally oriented transition dipole moments. Practically, an EQE of 40% is possible with q PL =0.95 and Θ=0.95. The value is significantly higher than that achievable with randomly oriented emitting dipoles. Materials Materials (>99%) were purchased from Furuya Metals (Tokyo, Japan) and Nichem Fine Technology Co., Ltd (Hsinchu County, Taiwan). The energy levels of the organic materials were obtained from the literature [1] , except for those of NPB. The HOMO level of NPB was measured using cyclic voltammetry. The LUMO level of NPB was estimated using the HOMO level and the optical band gap from its absorption spectrum. PL measurements PL spectra of the organic materials were measured using samples thermally deposited on fused silica under a vacuum of <5 × 10 −7 Torr. The samples were excited with a He/Cd laser (325 nm) to detect PL using a photomultiplier tube attached to a monochromator. Device fabrication The OLEDs were fabricated on clean glass substrates pre-patterned with 100-nm-thick ITO under a pressure of 5 × 10 −7 Torr by thermal evaporation without breaking the vacuum. Before the deposition of the organic layers, the ITO substrates were pre-cleaned with isopropyl alcohol and acetone, then exposed to ultraviolet-ozone for 10 min. The devices had the following layer structure: ITO (100 nm)/TAPC (75 nm)/NPB (10 nm)/NPB: B3PYMPM: red dopants [Ir (phq) 3 , Ir(mphq) 2 acac, Ir(MDQ) 2 acac, Ir(mphmq) 2 tmd] (30 nm, 3.5 mol%)/B3PYMPM (10 nm)/B3PYMPM:Rb 2 CO 3 (45 nm, 2 wt%)/Al (100nm). Each layer was deposited at a rate of 1 Å s −1 , and the deposition rate of the co-deposited layers was 1 Å s −1 in total. Device characterization The current densities, luminance intensities and EL spectra were measured using a programmable source meter (Keithley 2400) and a spectrophotometer (Spectrascan PR650, Photo Research). The angular distribution of the EL was measured with a programmable source meter (Keithley 2400), a goniometer, and a fibre optic spectrometer (Ocean Optics S2000). The EQE and the power efficiency of the OLEDs were calculated from their J – V – L characteristics, their EL spectra and the angular distribution of the EL intensity. Measurement and calculation of angle-dependent PL spectra The dipole orientations in the red dyes in the birefringent NPB:B3PYMPM co-host were determined by analysing the angle-dependent PL of the film using the classical dipole model [12] , [15] , [30] , [31] , [32] . This model allows for the separate calculation of the p - and s -polarized light emission from horizontally and vertically oriented dipoles in a non-absorbing anisotropic medium. According to the dipole model, the horizontally and vertically oriented dipoles, p x and p z , emit p -polarized light, whereas the other horizontally oriented dipole, p y , emits s -polarized light. The angle-dependent emission intensity of the p -polarized light is significantly different for the p x and p z dipoles, allowing the proportion of horizontal dipoles to be determined by fitting the simulated p -polarized intensity for various ratios of p x and p z to the experimental data. Using this method, the ratio of horizontal ( P ‖ = p x+ p y ) to vertical ( P ⊥ = p z ) dipoles can be evaluated. The refractive index of the optically anisotropic NPB:B3PYMPM layer was measured by VASE and is shown in Supplementary Fig. 1 . The incident angle was varied from 45° to 75° in steps of 5°. The experimental setup has been reported previously [12] , [15] and was composed of a motorized rotation stage, a half cylinder lens with a sample holder, a dichroic mirror to filter the excitation beam, a polarizer to select the polarization of the emitted light and a fibre optic spectrometer (Ocean Optics Maya2000). A He-Cd continuous wave laser (325 nm) was used as the excitation source. NPB:B3PYMPM films (30-nm thick) doped with 3.5 mol% red dye, which were thermally deposited on a 1-mm-thick fused silica substrate and encapsulated under N 2 atmosphere before use, were used for the angle-dependent PL measurements. P -polarized light was used to analyse the orientation of the dipoles in the films. Simulation of the outcoupling efficiency of the OLEDs The outcoupling efficiency of the devices was evaluated using the obtained dipole orientations. The device structure used to calculate the outcoupling efficiency was ITO (100 nm)/TAPC (75 nm)/NPB (10 nm)/NPB:B3PYMPM:Ir(mphmq) 2 tmd (30 nm)/B3PYMPM (x nm)/Al (100 nm). The thickness ( x nm) of the B3PYMPM layer was varied from 0 to 200 nm. The method has been described in detail elsewhere [4] , [32] . The refractive indices of the organic materials were measured by VASE, and those of ITO and Al were obtained from the literature [33] , [34] . The refractive index of the glass substrates (Corning Incorporated Eagle 2000) was taken from the manufacturer. The influence of the dopant on the refractive index of the EML was ignored because of the low doping concentration used. DFT/TD-DFT calculations on the iridium phosphorescent dyes Quantum chemical calculations based on DFT were carried out using Gaussian 09 programme [35] . An N , N -trans structure was used as the starting geometry. The ground-state and triplet-state geometry optimization were performed using Becke’s three-parameter B3LYP exchange–correlation functional [36] , [37] , [38] , the ‘double-ξ’ quality LANL2DZ basis set for the Ir atom, and the 6-311+G(d,p) basis set for all other atoms. A pseudo potential (LANL2DZ) was applied to replace the inner core electrons of the Ir atom, leaving the outer core [(5s)2(5p)6] electrons and the (5d)6 valence electrons. For the TD-DFT calculations, the unrestricted uB3LYP functional and the same basis sets used for geometry optimization were applied to the optimized geometry. The 20 lowest singlet and triplet states were calculated and analysed. The transition dipole moments of the triplet states were calculated using the Dalton 2011 programme with a quadratic response function and the 6-31G* basis set for C, H; the 6-311G* basis set for N, O; and the Stuttgart ECP basis set for Ir in the TD-DFT calculations. Structure optimization and the Kohn–Sham orbitals were calculated using the Gaussian 09 programme [35] , while the triplet transition dipole moments were calculated using the Dalton 2011 programme [25] . To efficiently identify the binding geometry between the host and the dopant, the calculations for the ESP map, which suggests plausible binding sites for the hosts and dopants by scanning the partial charge distributions on the molecular skeletons of each host and dopant molecule, were performed using the ESP method by Singh and Kollman [39] . The DFT geometry optimizations were then performed with the initial geometries, where the host and dopant were placed near the binding space suggested by the ESP map of each molecule. For the DFT computations, the Perdew–Burke–Ernzerhof [27] exchange–correlation functional was used using DMol3 in Materials Studio [40] , [41] . The electronic configurations were described by the double numerical basis set and the polarization basis set under an ECP. The optimization convergence thresholds for energy change, maximum force and maximum displacement were 0.00001 Ha, 0.002 Ha Å −1 and 0.005 Å, respectively. How to cite this article: Kim, K.-H. et al . Phosphorescent dye-based supramolecules for high-efficiency organic light-emitting diodes. Nat. Commun. 5:4769 doi: 10.1038/ncomms5769 (2014).